Spin-dependent charge transfer state design rules in organic photovoltaics Charge transfer states play a crucial role in organic photovoltaics, mediating both photocurrent generation and recombination losses. In this work, we examine recombination losses as a function of the electron-hole spacing in fluorescent charge transfer states, including direct monitoring of both singlet and triplet charge transfer state dynamics. Here we demonstrate that large donor–acceptor separations minimize back transfer from the charge transfer state to a low-lying triplet exciton ‘drain’ or the ground state by utilizing external pressure to modulate molecular spacing. The triplet drain quenches triplet charge transfer states that would otherwise be spin protected against recombination, and switches the most efficient origin of the photocurrent from triplet to singlet charge transfer states. Future organic solar cell designs should focus on raising the energy of triplet excitons to better utilize triplet charge transfer mediated photocurrent generation or increasing the donor–acceptor spacing to minimize recombination losses. Charge transfer (CT) states are bound combinations of an electron and a hole located on separate molecules [1] , [2] , [3] . They are formed on neighbouring molecules at donor–acceptor interfaces in organic photovoltaics (OPVs) after dissociation of excitons or during recombination of free charge [4] , [5] , [6] . Modern OPVs demonstrate ultrafast formation of CT states from excitons, and efficient dissociation of CT states into charge under short circuit conditions [7] . Indeed, internal quantum efficiencies of many OPVs now commonly approach 100% (ref. 8 ). But charge recombination losses mediated by CT states remain a problem in even the best devices [9] , [10] , [11] , [12] , [13] , increasing markedly at weaker internal electric fields, reducing open circuit voltage and power efficiency. Synthetic control over donor and acceptor OPV materials enables us to engineer the physical separation of the electron and hole at the donor–acceptor interface. This prompts an important question in OPV: What’s the effect of the CT state size? On one hand, separated CT states have smaller Coulombic binding energies, which should improve the photocurrent yield. But large separations are also expected to possess weaker coupling to the initial exciton, potentially reducing the exciton dissociation rate at donor–acceptor interfaces [14] . In addition, increased charge separation significantly reduces exchange splitting between singlet and triplet CT states. When the two are nearly degenerate, intersystem crossing between the two is fast, facilitating spin engineering that could improve the efficiency of OPVs. For example, spin-1 triplet CT states are forbidden from recombining to the ground state, which is typically a spin-0 singlet. Traditional OPV designs demand, however, that the CT state energy be as high as possible to maximize the open circuit voltage [15] , [16] . Typically, this pushes the CT energy above the energy of the triplet exciton on the donor or acceptor. As the lowest energy excited state in the system, the triplet exciton traps the energy originally contained in the CT state until it eventually recombines with the ground state, creating a crucial loss pathway or ‘triplet drain’ [3] , [10] . In the following, we characterize the complex set of tradeoffs for singlet and triplet CT states by applying external pressure to donor–acceptor blends [17] , [18] and observe its effect on the principal spin-dependent loss pathways ( Fig. 1 ). Singlet CT states recombine directly to the singlet ground state of the donor and acceptor, and we find that this loss pathway is exacerbated as the CT state is physically constrained. Applied pressure also enhances the back transfer from triplet CT states to low-lying triplet exciton drains present on either the donor or acceptor [9] , [13] . Applying a magnetic field to decrease the conversion of singlet CT states to triplet CT states allows us to identify the spin of the CT states responsible for the efficient generation of photocurrent. We find that when a triplet drain is present, singlet CT states are responsible for the efficient generation of photocurrent, but in the absence of a triplet drain, photocurrent is more efficiently generated from the triplet CT states. Consequently, we find that the CT states of conventional OPVs should be designed to be as physically large as possible, to minimize the back transfer from triplet CT states to triplet excitons, and with minimal sources of spin mixing within the CT manifold, to prevent intersystem crossing from the original singlet CT state. In the absence of low-lying triplet excitons, however, we find that triplet CT states are the most efficient source of photocurrent because they are spin protected against recombination. Devices without triplet drains tolerate compressed CT states, even showing extended CT state lifetimes under applied pressure. 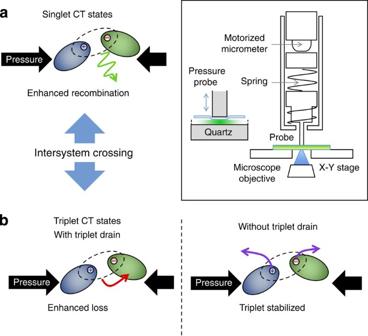Figure 1: Schematic of charge transfer state dynamics and pressure setup. Schematic of expected changes in (a) singlet and (b) triplet charge transfer (CT) states as a function of their size. The possible triplet dynamics are dependent on the presence of a triplet quenching state or ‘drain’ on the donor or the acceptor. (inset) The measurement apparatus used to apply pressure to the films. Figure 1: Schematic of charge transfer state dynamics and pressure setup. Schematic of expected changes in ( a ) singlet and ( b ) triplet charge transfer (CT) states as a function of their size. The possible triplet dynamics are dependent on the presence of a triplet quenching state or ‘drain’ on the donor or the acceptor. (inset) The measurement apparatus used to apply pressure to the films. Full size image Charge transfer state dynamics Singlet and triplet CT states are monitored as a function of size using a set of exciplex emitters originally designed for thermally activated delayed fluorescence (TADF) in organic light-emitting devices. Two specific TADF thin film blends were selected: 4,4′,4″-tris[3-methylphenyl(phenyl)amino]triphenylamine (m-MTDATA) as the donor and either tris-[3-(3-pyridyl)mesityl]borane (3TPYMB) or 2-(biphenyl-4-yl)-5-(4-tert-butylphenyl)-1,3,4-oxadiazole (t-Bu-PBD) as the acceptor ( Fig. 2a ). See Methods for sample and device fabrication. These materials have been demonstrated to fluoresce from the exciplex CT state with efficiencies of ~20% and they exhibit the bi-exponential transient fluorescence decays and temperature-dependence characteristic of single-molecule TADF emitters [19] . 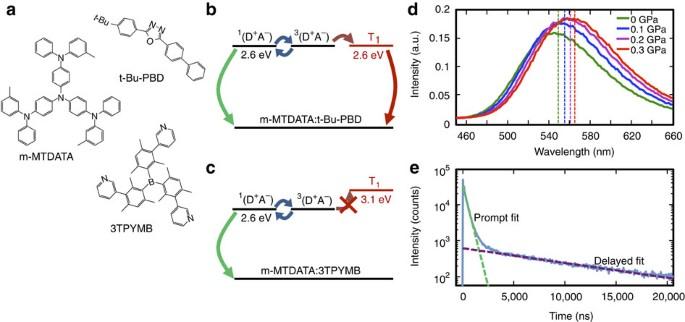Figure 2: Material systems and charge transfer state characterization. (a) Chemical structures of m-MTDATA, t-Bu-PBD and 3TPYMB. (b) The crucial energy levels and rates for the m-MTDATA:t-Bu-PBD and (c) m-MTDATA:3TPYMB systems. The excitonic triplet state T1state is for the acceptor; the excitonic triplet of m-MTDATA is ~2.7 eV (not shown). (d) Measured m-MTDATA:3TPYMB film PL under pressure. Vertical line indicates the peak wavelength. (e) Transient PL for the m-MTDATA:t-Bu-PBD system. Green and purple dashed lines indicate fitted prompt and delay lifetimes, respectively. Figure 2: Material systems and charge transfer state characterization. ( a ) Chemical structures of m-MTDATA, t-Bu-PBD and 3TPYMB. ( b ) The crucial energy levels and rates for the m-MTDATA:t-Bu-PBD and ( c ) m-MTDATA:3TPYMB systems. The excitonic triplet state T 1 state is for the acceptor; the excitonic triplet of m-MTDATA is ~2.7 eV (not shown). ( d ) Measured m-MTDATA:3TPYMB film PL under pressure. Vertical line indicates the peak wavelength. ( e ) Transient PL for the m-MTDATA:t-Bu-PBD system. Green and purple dashed lines indicate fitted prompt and delay lifetimes, respectively. Full size image The dynamics of both the systems are shown in the rate diagrams of Fig. 2b,c . Three critical states define the system: singlet CT state 1 (D + A − ), triplet CT state 3 (D + A − ) and excitonic triplet states. In both the systems, the singlet CT state lies at ~2.6 eV as determined by exciplex CT state fluorescence. The triplet CT state is nearly isoenergetic with the singlet CT state; the triplet CT for the t-Bu-PBD acceptor system is estimated to be between 5 and 50 meV lower than that of the singlet CT state [19] , [20] . Note that the observed CT state emission in these systems is due to the exciplex singlet CT state between the nearest neighbor donor–acceptor molecules. Spin-orbit coupling-induced intersystem crossing (ISC) and reverse intersystem crossing modulates the interaction between singlet and triplet exciplex CT states. In addition, donor/acceptor systems like this may also contain another intersystem crossing mechanism, in which temporary delocalization of a CT state to form a polaron pair results in degeneracy of the singlet and triplet states, which are then interconverted through hyperfine coupling with the local magnetic nuclei. This mechanism is affected by an external magnetic field, as will be discussed below [21] , [22] , [23] , [24] . To eliminate complications from potential interactions with m-MTDATA excimers [20] , we focus on the relative changes incurred when the acceptor changes from 3TPYMB to t-Bu-PBD while maintaining a constant fraction of the m-MTDATA donor molecules. Of particular importance to these systems are the excitonic triplet energies. The m-MTDATA triplet exciton lies at 2.7 eV [19] , and is therefore uphill from the triplet CT state. The 3TPYMB triplet exciton lies at ~3.1 eV and is energetically inaccessible from the triplet CT state, effectively preventing the back transfer to a triplet drain on 3TPYMB. In contrast, the t-Bu-PBD triplet exciton lies at 2.6 eV (ref. 25 ) or below ( Supplementary Fig. 1 , Supplementary Note 1 ), approximately isoenergetic with the m-MTDATA:t-Bu-PBD CT state. Thus, the triplet back transfer is blocked in the m-MTDATA:3TPYMB system due to the high energies of the triplet excitons, while the m-MTDATA:t-Bu-PBD system has potentially significant triplet back transfer. Since modern OPVs typically possess triplet drains, the t-Bu-PBD system may be a closer analogue for conventional high-efficiency devices. Pressure effect measurements Pressure effect measurements were performed using mechanical setup shown in Fig. 1 inset (see Methods). As expected, emission from the exciplex CT state in a blended film quenches both exciton fluorescence and phosphorescence from the donor and acceptor materials [19] . Figure 2d demonstrates the effects of pressure on steady-state photoluminescence (PL) of the CT state emission. Increasing external pressure leads to a red shift in emission energy. The red shift is due to both solvation effect from increased molecular density and increased Coulomb interaction between the donor and acceptor in the compressed geometry [26] , [27] . A significant increase in fluorescence intensity was also observed ( Supplementary Fig. 2 , Supplementary Note 2 ). To better understand the dynamics of the system, we measured time-resolved fluorescence using time-correlated single-photon detector. Figure 2e illustrates a typical transient PL measurement under no external pressure. It is evident that there are distinct prompt and delayed dynamics in the system. We define the prompt emission to be within the first 0.3–0.7 μs and delayed emission to be between 4–9 μs for m-MTDATA:t-Bu-PBD and 8–12 μs for m-MTDATA:3TPYMB ( Supplementary Fig. 3 , Supplementary Note 3 ). Following Goushi et al . [19] , we attribute the prompt emission to singlet CT states and the delayed emission to dynamics of triplet CT states. We fit a single exponential to each of these time windows and compare the pressure-dependent transient dynamics of m-MTDATA:t-Bu-PBD and m-MTDATA:3TPYMB. This reveals the effect of the low-lying t-Bu-PBD triplet exciton drain on the dynamics of singlet and triplet CT states. As the molecules are pushed closer together, the red shift in the emission spectrum suggests that the overlap between the donor HOMO and acceptor LUMO increases, with significant additional consequences for the photophysics. Recombination processes back to localized states increase—most notably fluorescence from the singlet CT state due to an increase in the transition dipole moment. We also expect both the forward and reverse intersystem crossing rates to slow for CT states localized on neighbouring molecules; the exchange splitting is proportional to the overlap of the donor HOMO and the acceptor LUMO and therefore will increase under pressure, and to the first order, the mixing between triplet and singlet states is inversely proportional to the exchange splitting. The trends in prompt dynamics under pressure are shown in Fig. 3 , with the transient lifetime and intensity data plotted in Fig. 3a,b , respectively. A large increase in prompt intensity is observed in both the material systems. The accompanying prompt lifetime change is determined by the competition between a decrease in the ISC rate and an increase in fluorescence rate. Indeed, for the m-MTDATA:t-Bu-PBD system, we see little change in the overall lifetime, reflecting that the increase in recombination rate is offset by the decrease in ISC rate. However, a similar prompt lifetime measurement of the m-MTDATA:3TPYMB system shows that the increase in recombination rate dominates the decrease in ISC rate. 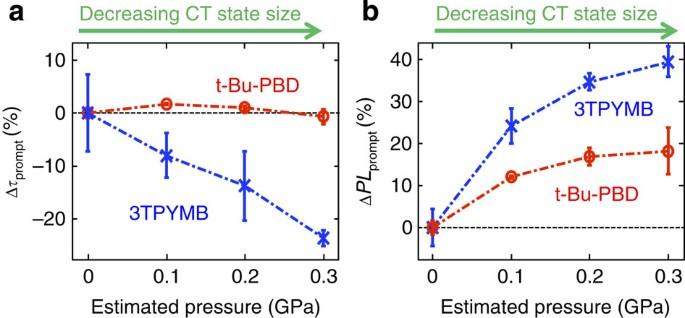Figure 3: Pressure effect on prompt charge transfer emission. (a) Prompt lifetime and (b) integrated prompt intensity changes with applied pressure for the two exciplex systems, where prompt emission is defined as 0.3–0.7 μs after excitation. Blue data points are from the m-MTDATA:3TPYMB system; red are from m-MTDATA:t-Bu-PBD. Error bars are calculated using s.d. of six independent measurements at each pressure to indicate measurement variations. Figure 3: Pressure effect on prompt charge transfer emission. ( a ) Prompt lifetime and ( b ) integrated prompt intensity changes with applied pressure for the two exciplex systems, where prompt emission is defined as 0.3–0.7 μs after excitation. Blue data points are from the m-MTDATA:3TPYMB system; red are from m-MTDATA:t-Bu-PBD. Error bars are calculated using s.d. of six independent measurements at each pressure to indicate measurement variations. Full size image The trends in delayed dynamics under pressure are shown in Fig. 4 . The delayed dynamics, which primarily reflect the dynamics of triplet CT states, show significant deviation between the two material systems. In the m-MTDATA:3TPYMB system, the probability of back transfer to a molecular triplet exciton is small, thus, an increase in delayed lifetime is observed due to the reduced rate of reverse intersystem crossing. The effect of changes in the exchange splitting is insignificant to the intensity of integrated delayed emission, which still tracks the change in prompt intensity and radiative rate. In the m-MTDATA:t-Bu-PBD system, by contrast, increasing the pressure significantly decreases the delayed lifetime and intensity. We attribute this to an increase in triplet back transfer loss: the exciplexes are drained through this loss channel due to better coupling with the localized t-Bu-PBD triplet (reflected in the decreased lifetime). Thus, triplet back transfer is a significant loss mechanism in the m-MTDATA:t-Bu-PBD system that only worsens as the spacing between the electron and the hole decreases. 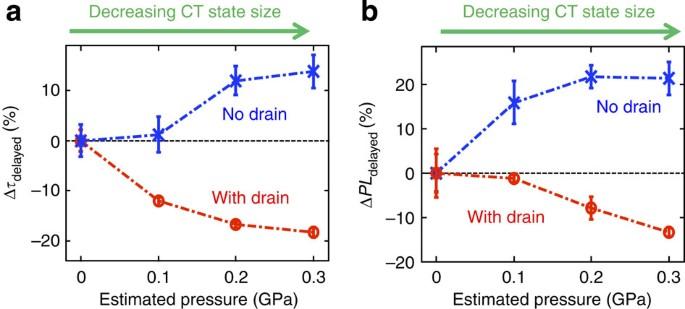Figure 4: Pressure effect on delayed charge transfer emission. (a) Delayed lifetime and (b) integrated delayed intensity changes with applied pressure for the two exciplex systems. Blue data points are from the m-MTDATA:3TPYMB system, where delayed emission is defined to be in the time span of 8–12 μs after excitation; red data points are from m-MTDATA:t-Bu-PBD, where delayed emission is defined to be in the time span of 4–9 μs after excitation. The delayed fluorescence quenching with increasing pressure in m-MTDATA:t-Bu-PBD clearly indicates triplet back transfer to a triplet drain. Error bars are calculated using s.d. of six independent measurements at each pressure to indicate measurement variations. Figure 4: Pressure effect on delayed charge transfer emission. ( a ) Delayed lifetime and ( b ) integrated delayed intensity changes with applied pressure for the two exciplex systems. Blue data points are from the m-MTDATA:3TPYMB system, where delayed emission is defined to be in the time span of 8–12 μs after excitation; red data points are from m-MTDATA:t-Bu-PBD, where delayed emission is defined to be in the time span of 4–9 μs after excitation. The delayed fluorescence quenching with increasing pressure in m-MTDATA:t-Bu-PBD clearly indicates triplet back transfer to a triplet drain. Error bars are calculated using s.d. of six independent measurements at each pressure to indicate measurement variations. Full size image Magnetic field effect measurements Next we probe the CT state populations and resulting changes in photocurrent by applying an external magnetic field to the device and simultaneously monitoring fluorescence and photocurrent [21] . The magnetic fields used in this experiment split two of the three triplet levels by up to~50 μeV. This Zeeman splitting is inconsequential to the intersystem crossing between the tightly bound CT states, because the exchange splitting between the singlet and triplet states is much larger than 50 μeV. Instead, the magnetic field only modulates intersystem crossing between singlet and triplet states of larger CT states (PPs) whose exchange splitting is much <~50 μeV. Indeed, as noted by Frankevich, et al . [22] , the magnetic field effect is due to an initial population of singlet CT states that temporarily separate beyond their exchange radius, forming Coulombically bound polaron pair states with zero effective exchange splitting. Such an extended singlet state may undergo intersystem crossing to a triplet mediated by hyperfine interactions. Otherwise, if the state remains as a singlet, it may collapse back and radiatively recombine within the spin-relaxation time [21] , [22] , [23] , [24] . Therefore, we expect the magnetic field-induced increase in the probability of geminately recombining to singlet CT state to lead to an increase in the fluorescence quantum yield. Indeed, an increase in fluorescence under magnetic field was observed in both the material systems; see Fig. 5a . 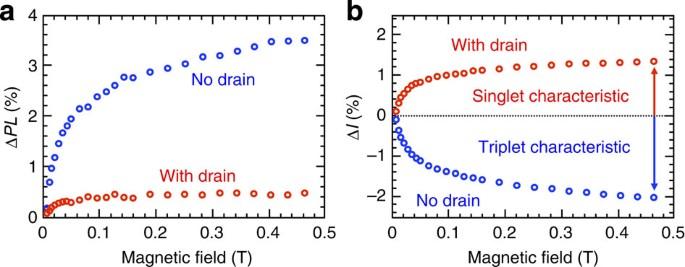Figure 5: Magnetic field effect on fluorescence and photocurrent. (a) Magnetic field effect on fluorescence for the m-MTDATA:t-Bu-PBD (red) and m-MTDATA:3TPYMB (blue) systems. Increases in PL from both the systems demonstrate that the applied magnetic field increases the population of singlet CT states. (b) The magnetic field effect on photocurrent for the m-MTDATA:t-Bu-PBD (red) and m-MTDATA:3TPYMB (blue) systems. The positive magnetic field effect with the t-Bu-PBD acceptor indicates that current is most efficiently collected from the singlet CT state, while the negative magnetic field effect with the 3TPYMB acceptor indicates that current is more efficiently collected from the triplet CT state. Figure 5: Magnetic field effect on fluorescence and photocurrent. ( a ) Magnetic field effect on fluorescence for the m-MTDATA:t-Bu-PBD (red) and m-MTDATA:3TPYMB (blue) systems. Increases in PL from both the systems demonstrate that the applied magnetic field increases the population of singlet CT states. ( b ) The magnetic field effect on photocurrent for the m-MTDATA:t-Bu-PBD (red) and m-MTDATA:3TPYMB (blue) systems. The positive magnetic field effect with the t-Bu-PBD acceptor indicates that current is most efficiently collected from the singlet CT state, while the negative magnetic field effect with the 3TPYMB acceptor indicates that current is more efficiently collected from the triplet CT state. Full size image However, there is a striking difference between these material systems when we examine the magnetic field effect on photocurrent measured simultaneously with the fluorescence in Fig. 5b . In the m-MTDATA:t-Bu-PBD system, the magnetic field effect on the photocurrent is also positive, that is, as the singlet CT population increases with the applied field, the photocurrent simultaneously increases. This signifies that the photocurrent is more efficiently generated from the singlet CT state, confirming our observation of significant back transfer loss processes quenching the triplet CT states in this material system. Photocurrent from the m-MTDATA:3TPYMB system, however, shows the opposite effect, decreasing with applied magnetic field. As the singlet CT population increases with an applied external magnetic field the triplet CT population must correspondingly decrease. Because the change in the photocurrent is negative with increasing applied field, we conclude that photocurrent must be more effectively collected through the triplet CT state in the m-MTDATA:3TPYMB system. Indeed, given the dependence of its triplet CT state lifetime on pressure, the magnetic field effect suggests that m-MTDATA:3TPYMB is spin protected in the triplet state. This direct measurement of CT state fluorescence and photocurrent generation under magnetic field indicates that triplet CT is more efficient in photocurrent generation in this system, since recombination to the ground state is spin forbidden, and recombination to a triplet exciton is energetically unfavourable. These results are reminiscent of recent studies of the P3HT:PCBM OPV system, where alternative methods showed evidence that the spin protection of triplet CT states can lead to longer lifetimes and greater probability of dissociation to free charges [28] , [29] . We also note that there was no measurable magnetic field effect on dark conductivity of our devices, indicating the absence of complicating magnetoresistance phenomena. Finally, we examine the effects on actual device performance in Fig. 6 . Drastic performance reduction due to triplet back transfer is readily apparent in m-MTDATA:t-Bu-PBD. Allowing the triplet CT state to generate photocurrent in the m-MTDATA:3TPYMB system that is associated with a factor of four increase in peak external quantum efficiency as compared with the t-Bu-PBD system, demonstrating the necessity of minimizing triplet back transfer in future photovoltaic material designs and the potential benefits of spin-protected triplet CT states. In Fig. 6b we show that open circuit voltage of m-MTDATA:3TPYMB is significantly higher than that of m-MTDATA:t-Bu-PBD, demonstrating that the decrease in recombination losses resulting from spin protection in the absence of a triplet drain is preserved at weaker internal electric fields. 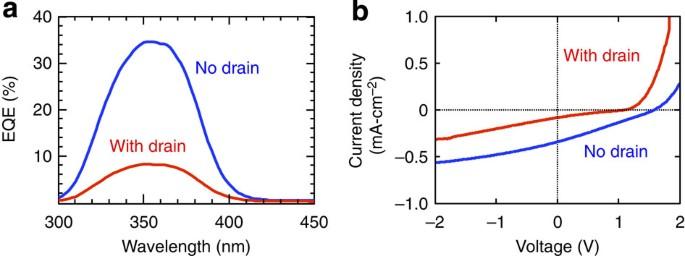Figure 6: Photovoltaic device characteristics. (a) External quantum efficiencies of m-MTDATA:3TPYMB (blue) and m-MTDATA:t-Bu-PBD blends (red). Triplet back transfer to the triplet drain on t-Bu-PBD is associated with decreased efficiency relative to the 3TPYMB system. (b) Current-voltage curves for the m-MTDATA:3TPYMB (blue) and m-MTDATA:t-Bu-PBD blends (red). Turning off the triplet drain correlates with a large increase in open circuit voltage. Figure 6: Photovoltaic device characteristics. ( a ) External quantum efficiencies of m-MTDATA:3TPYMB (blue) and m-MTDATA:t-Bu-PBD blends (red). Triplet back transfer to the triplet drain on t-Bu-PBD is associated with decreased efficiency relative to the 3TPYMB system. ( b ) Current-voltage curves for the m-MTDATA:3TPYMB (blue) and m-MTDATA:t-Bu-PBD blends (red). Turning off the triplet drain correlates with a large increase in open circuit voltage. Full size image Open circuit voltage maximization in OPVs typically requires that CT states be as high in energy as possible—higher, in fact, than the triplet exciton. [15] , [16] Under this constraint, our work demonstrates the ability to reduce CT state recombination and back transfer losses by maximizing the electron-hole spacing at the interface. The optimum size of the CT state then occurs when the formation rate of the CT state from the molecular exciton is on the order of the excitonic recombination loss rate. Our results also indicate that the current paradigm regarding the necessity of maximal-energy CT states may not be as absolute as it is currently believed to be. Substantial benefits in both EQE and open circuit voltage were shown to result from the spin protection of triplet CT states when the exciton triplet energy is high enough to cutoff back transfer to triplet excitons. Ideal OPV materials, instead, may look more like inorganic quantum dots or organic light-emitting device TADF materials, with minimal Stokes shift and negligible splitting between the singlet and triplet states [30] . The absence of a triplet drain in these systems should allow some CT states to be spin protected from recombination, a property that may be unique to excitonic solar cell materials. Sample fabrication To characterize CT state dynamics of m-MTDATA:3TPYMB and m-MTDATA:t-Bu-PBD we deposited thin films for pressure testing and made OPV devices to obtain the magnetic field dependence of photocurrent. OPV devices consisted of 60 nm of a 1:1 molar donor–acceptor blend thermally evaporated on 15 ohms per square ITO and capped with 100 nm of aluminium. All organic materials were purchased from Lumtec (Luminescence Technology Corp.) and used as received. The blended heterojunction films for pressure testing consisted of 60 nm of a 1:1 molar blend thermally evaporated on thick glass samples with 100 nm of aluminium deposited on the top of the blend for consistency in reflection under pressure. The samples were then encapsulated with thin flexible glass covers and epoxy. Pressure measurements Pressure was applied using a motorized micrometre system with known force through a probe; see Fig. 1 (inset). The applied force distorts the substrate, and we estimated the contact area (radius ~100 μm) to obtain the applied pressure on the film through the top flexible cover glass. Optical characterization was performed through the substrate using a microscope setup with a λ=405 nm pulsed 31.25 kHz excitation laser (PicoQuant LDH) focused to ~10 μm spot size. A 405 nm dichroic and a 450-nm long-pass filter was used to filter CT state emissions. A spectrometer (Princeton Instrument Acton) was used to take steady-state PL measurements. Time-resolved PL measurements were taken using an avalanche photodiode single-photon detector (PicoQuant PDM). Magnetic field measurements Measurements of the change in photocurrent or fluorescence with magnetic field were performed following the procedure described in Congreve et al . [31] , using monochromatic 365 nm light generated by an LED that was mechanically chopped. An electromagnet applied the magnetic field at a frequency of 13 mHz with a duty cycle of 50%. The fluorescence was captured by a silicon photodetector and measured by a lock-in amplifier. The device photocurrent was simultaneously captured by a second lock-in. The magnetic field was measured by an FWBell 5100 gaussmeter. Both the readings were queried at a frequency of 1 Hz. How to cite this article: Chang, W. et al . Spin-dependent charge transfer state design rules in organic photovoltaics. Nat. Commun . 6:6415 doi: 10.1038/ncomms7415 (2015).